CAND1 controlsin vivodynamics of the cullin 1-RING ubiquitin ligase repertoire The combinatorial architecture of cullin 1-RING ubiquitin ligases, in which multiple F-box containing substrate receptors compete for access to CUL1, poses special challenges to assembling cullin 1-RING ubiquitin ligase complexes through high affinity protein interactions while maintaining the flexibility to dynamically sample the entire F-box containing substrate receptor repertoire. Here, using highly quantitative mass spectrometry, we demonstrate that this problem is addressed by CAND1, a factor that controls the dynamics of the global cullin 1-RING ubiquitin ligase network by promoting the assembly of newly synthesized F-box containing substrate receptors with CUL1-RBX1 core complexes. Our studies of in vivo cullin 1-RING ubiquitin ligase dynamics and in vitro biochemical findings showing that CAND1 can displace F-box containing substrate receptors from Cul1p suggest that CAND1 functions in a cycle that serves to exchange F-box containing substrate receptors on CUL1 cores. We propose that this cycle assures comprehensive sampling of the entire F-box containing substrate receptor repertoire in order to maintain the cullin 1-RING ubiquitin ligase landscape, a function that we show to be critical for substrate degradation and normal physiology. Cullin 1-RING ubiquitin ligases (CRL1s) are multifunctional ubiquitin ligases that uniquely exploit combinatorial diversity in order to achieve unparalleled versatility in substrate targeting and control of cell physiology [1] , [2] , [3] . This combinatorial layout where multiple F-box containing substrate receptors (FBPs) compete for access to CUL1 poses special challenges to assembling CRL1 complexes through high affinity protein interactions while maintaining the flexibility to dynamically sample the entire FBP repertoire. Mounting evidence has implicated mechanisms related to the reversible modification of CUL1 with the ubiquitin-related peptide NEDD8 in this regulation [4] , but no definitive model has been substantiated experimentally. Conjugation of NEDD8 to CUL1 stimulates the ubiquitin ligase activity of CRL1s [5] , [6] , and deneddylation by the COP9 signalosome resets CRL1s into an inactive state [7] , [8] , [9] . Deneddylation has two important consequences: it prevents the autocatalytic destruction of FBPs [10] , [11] , [12] and it allows CUL1 to associate with CAND1, a highly conserved protein that inhibits CUL1 neddylation and hence CRL1 activity in vitro [13] , [14] , [15] , [16] , [17] , [18] . This inhibition can be overcome by purified SKP1-FBP heterodimers, which dissociate the CUL1-CAND1 complex in vitro [18] , [19] . Paradoxically, however, CAND1 was also shown to promote CRL function in vivo [12] , [14] , [20] , [21] , [22] , [23] . In pursuit of this paradox, we previously showed that fission yeast cells deleted for knd1 , the orthologue of human CAND1, display an imbalance in CRL complexes formed between Cul1p and two epitope-tagged FBPs, Pof1p-Myc and Pof3p-Myc [12] . Whereas CRL1 Pof1p-Myc complexes increased, CRL1 Pof3p-Myc complexes were depleted in cells lacking knd1 . The ~2-fold decrease in the CRL1 Pof3p-Myc complex was sufficient to cause phenotypic defects that mirrored a Δ pof3 deletion mutant [12] , [24] , a finding that reinforced a positive role of CAND1/Knd1p in CRL1 control. Similar imbalances were reported for CUL1-TIR1 interactions in A. thaliana and for CUL3-KEAP1 interactions in human cells [25] , [26] . The latter studies also demonstrated that substrate degradation by CRL1 TIR1 and CRL3 KEAP1 is compromised either in the absence of CAND1 or when CAND1 is overexpressed. Based on these findings, we proposed that a CAND1-mediated cycle of CRL1 complex disassembly and subsequent reassembly maintains the cellular balance of CRL1 complexes and optimal CRL1 activity [12] . However, a subsequent study using siRNA-mediated knockdown in human cells achieved a partial reduction in CUL1-CAND1 complex but observed no significant effect on the recruitment of SKP1 (and presumably FBPs) to CUL1 and, therefore, relinquished a role of CAND1 in CRL1 assembly and remodelling [27] . We have used highly quantitative mass spectrometry to rigorously assess the impact of complete genetic depletion of CAND1/Knd1p on the global CRL1 repertoire and its assembly/disassembly dynamics. We demonstrate that CAND1/Knd1p has a crucial role in maintaining a balanced repertoire through mechanisms that are consistent with our previously proposed CAND1 cycle [12] . CAND1/Knd1p maintains the global CRL1 repertoire To test the effect of complete genetic ablation of CAND1 on the native CRL1 repertoire, we immunopurified Cul1p-associated proteins from wild-type and Δ knd1 fission yeast cells differentially labelled with stable isotopes [28] and quantified them by liquid chromatography and tandem mass spectrometry (LC-MS/MS). Whereas Δ knd1 cells were grown in medium containing regular ammonium- 14 N chloride as the nitrogen source, the wild-type cells were metabolically labelled with ammonium- 15 N chloride with an efficiency of >98%. Cultures were mixed at a ratio of 1:1 and processed as a single sample for lysate preparation, Cul1p immunopurification and LC-MS/MS to quantify the relative abundance of Cul1p-associated proteins in wild-type and Δ knd1 cells based on averaged 14 N/ 15 N peptide ratios ( Fig. 1a ). Triplicate experiments revealed statistically significant ( P ≤0.05) differences in Cul1p occupancy by various FBPs. While occupancy by Pof1p, Pof7p, Pof9p, Pof10p and Pof14p increased by 1.3- to 2.2-fold, occupancy by Pof5p, Pof11p, Pof15p and Pop1p decreased by factors of 1.5- to 5-fold ( Fig. 1b ; Supplementary Table S1 ; Supplementary Data 1 ). The modest amplitude of these changes is explained by the fact that ~50% of Cul1p is neddylated in cells [10] . As neddylated Cul1p cannot interact with CAND1, this fraction of CRL1 complexes is not responsive to the cellular CAND1 status. 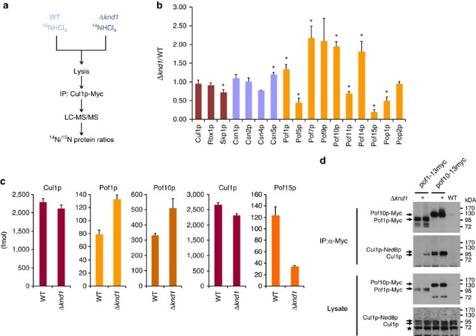Figure 1: Effect of Knd1p on the CRL1 repertoire. (a) Wild-type (WT)S. pombecells and cells deleted forknd1(Δknd1), which also carry a Myc-tagged allele of endogenous Cul1p, were grown in medium containing either ammonium-14N chloride or ammonium-15N chloride as the nitrogen sources. Equal numbers of cells were mixed at a ratio of 1:1, followed by the isolation of CRL1 complexes through immunopurification (IP) of Cul1p-Myc. The purified material was analysed by LC-MS/MS to identify Cul1p-associated proteins and to quantify their relative abundance in WT and Δknd1samples based on14N/15N peptide/protein ratios. (b) Relative abundance of Cul1p and Cul1p-interacting proteins in WT versus Δknd1cells. Triplicate data sets (Supplementary Data File 1) were averaged and s.d. values are indicated. Statistically significant changes (t-test,P≤0.05) are indicated by asterisks. (c) Absolute amounts of Cul1p, Pof1p and Pof10p retrieved from a 1:1 mixture of15N-labelled WT and14N-labelled Δknd1cells by Cul1p IP and mass spectrometry-based quantification by selected ion monitoring. The right hand panel shows the same measurements for Cul1p and Pof15p from an independent Cul1p IP sample. (d) Lysate of WT and Δknd1cells expressing Pof1p or Pof10p tagged with the c-Myc epitope were used in immunoprecipitation with anti-Myc antibodies, followed by detection of co-precipitated proteins with either anti-Myc or anti-Cul1p antibodies. The neddylated and unneddylated forms of Cul1p are indicated. Total cell lysate is shown in the bottom two panels. The asterisk denotes a crossreactivity of the anti-Cul1p antibody. Figure 1: Effect of Knd1p on the CRL1 repertoire. ( a ) Wild-type (WT) S. pombe cells and cells deleted for knd1 (Δ knd1 ), which also carry a Myc-tagged allele of endogenous Cul1p, were grown in medium containing either ammonium- 14 N chloride or ammonium- 15 N chloride as the nitrogen sources. Equal numbers of cells were mixed at a ratio of 1:1, followed by the isolation of CRL1 complexes through immunopurification (IP) of Cul1p-Myc. The purified material was analysed by LC-MS/MS to identify Cul1p-associated proteins and to quantify their relative abundance in WT and Δ knd1 samples based on 14 N/ 15 N peptide/protein ratios. ( b ) Relative abundance of Cul1p and Cul1p-interacting proteins in WT versus Δ knd1 cells. Triplicate data sets ( Supplementary Data File 1 ) were averaged and s.d. values are indicated. Statistically significant changes ( t -test, P ≤0.05) are indicated by asterisks. ( c ) Absolute amounts of Cul1p, Pof1p and Pof10p retrieved from a 1:1 mixture of 15 N-labelled WT and 14 N-labelled Δ knd1 cells by Cul1p IP and mass spectrometry-based quantification by selected ion monitoring. The right hand panel shows the same measurements for Cul1p and Pof15p from an independent Cul1p IP sample. ( d ) Lysate of WT and Δ knd1 cells expressing Pof1p or Pof10p tagged with the c-Myc epitope were used in immunoprecipitation with anti-Myc antibodies, followed by detection of co-precipitated proteins with either anti-Myc or anti-Cul1p antibodies. The neddylated and unneddylated forms of Cul1p are indicated. Total cell lysate is shown in the bottom two panels. The asterisk denotes a crossreactivity of the anti-Cul1p antibody. Full size image To corroborate these data, we performed a control experiment to exclude that CRL1 complexes rearrange during the immunopurification from mixed 14 N and 15 N cell lysates. For this, we mixed equal parts of 15 N-labelled lysate from wild-type cells carrying a Cul1p-Myc allele with unlabelled lysate of Δ knd1 cells lacking a Cul1p-Myc allele. When Cul1p complexes were purified and analysed by LC-MS/MS, CRL1 components were almost exclusively represented by 15 N peptides ( Supplementary Fig. S1a,b ). This finding indicates that 14 N-labelled subunits present in the lysate of untagged cells did not enter CRL1 complexes at an appreciable rate after cell lysis. In contrast, proteins that were unspecifically retrieved on the beads were represented by both 14 N and 15 N peptides at roughly equal parts ( Supplementary Fig. S1b ). We subsequently applied LC-MS/MS-based absolute protein quantification technology using isotopically labelled reference peptides (absolute quantification (AQUA) [29] to measure the exact amounts of FBPs retrieved in CRL1 complexes. In agreement with the relative quantification data, the absolute amounts of Pof1p and Pof10p were 1.5–1.7-fold higher in complexes isolated from Δ knd1 cells than from wild-type cells ( Fig. 1c ; Supplementary Data 2 ). While 3.5% of Cul1p was occupied by Pof1p in wild-type cells, the fraction increased to 6.2% in Δ knd1 cells ( Supplementary Data 2 ). Likewise, Cul1p occupancy by Pof10p increased from 14.5% to 24% in Δ knd1 cells. These increases were confirmed by reciprocal immunoprecipitation/immunoblotting experiments ( Fig. 1d ; Supplementary Fig. S1c ). Conversely, Pof15p levels were 3.5-fold lower in Cul1p complexes isolated from Δ knd1 cells ( Fig. 1c ) and the fractional occupancy for this FBP was reduced from 4.6% to 1.5% ( Supplementary Data 2 ). Again these absolute measurements confirmed the relative quantifications ( Fig. 1b ). The observed changes in Cul1p-FBP interactions are not due to concordant changes in steady-state FBP levels in Δ knd1 cells ( Fig. 2a ; ref. 12 ). Likewise, CRL1 core subunits Cul1p and Rbx1p were retrieved in equal amounts from both wild-type and Δ knd1 cells ( Fig. 1b ). Skp1p protein levels were ~40% higher in the mutant as determined by immunoblotting and quantitative mass spectrometry ( Fig. 2a ). Nevertheless, binding of Skp1p to Cul1p was decreased by ~25% in Δ knd1 cells ( Fig. 1b ). This finding, which contrasts with previous measurements in human cells showing that binding of SKP1 to CUL1 is slightly increased upon acute knockdown of CAND1 [13] , [14] , [27] , was highly reproducible across 179 individual Skp1p peptide measurements by LC-MS/MS ( Supplementary Data 3 ). It, therefore, appears that Schizosaccharomyces pombe cells devoid of Knd1p activity might have a ~25% overall reduction in fully assembled CRL1 complexes. The complexes that are assembled, however, dramatically differ in FBP composition relative to wild-type cells. 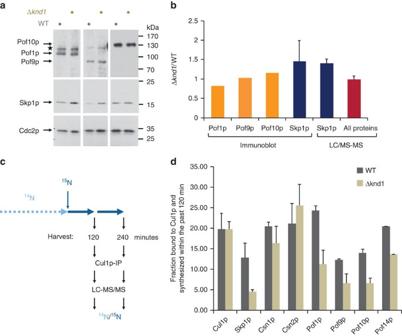Figure 2: Effect of Knd1p on CRL1 dynamics. (a) Steady-state levels of FBPs in wild-type (WT) and Δknd1cells. The expression of Pof1p, Pof9p and Pof10p modified with c-Myc epitopes at the endogenous genomic locus was determined by immunoblotting with Myc antibodies. Blots were reprobed with anti-Skp1p and anti-Cdc2p (PSTAIRE) antibodies as a reference. (b) The first three bars show a quantification of the FBP ratios in Δknd1versus WT cells apparent from the immunoblots inaas determined by film densitometry. Ratios are from values normalized to Cdc2p. The fourth bar shows the average Skp1p ratio obtained from four independent immunoblot measurements including s.d. The fifth bar shows the Δknd1/WT ratio of Skp1p quantified by LC-MS/MS. Skp1p was immunopurified independently four times from 1:1 mixtures of15N (WT) and14N (Δknd1) labelled cells. The average ratio and the s.d. were plotted. The sixth bar shows the average ratio of all proteins identified in the Skp1p purification. The ratio of these background proteins was close to 1.0 with a narrow s.d., supporting the significance of the ~1.5-fold increase in Skp1p levels in Δknd1cells. (c) Schematic outline of the15N pulse labelling strategy. Cells maintained in routine14N media were shifted to15N media for 120 or 240 min before the preparation of cell lysate, Cul1p IP and analysis by LC-MS/MS. (d) Relative fractions of newly synthesized FBPs and COP9 signalosome (CSN) subunits associated with Cul1p in wild-type and Δknd1cells. Data represent averages and s.d. values of three independent experiments (seeSupplementary Data 4). Figure 2: Effect of Knd1p on CRL1 dynamics. ( a ) Steady-state levels of FBPs in wild-type (WT) and Δ knd1 cells. The expression of Pof1p, Pof9p and Pof10p modified with c-Myc epitopes at the endogenous genomic locus was determined by immunoblotting with Myc antibodies. Blots were reprobed with anti-Skp1p and anti-Cdc2p (PSTAIRE) antibodies as a reference. ( b ) The first three bars show a quantification of the FBP ratios in Δ knd1 versus WT cells apparent from the immunoblots in a as determined by film densitometry. Ratios are from values normalized to Cdc2p. The fourth bar shows the average Skp1p ratio obtained from four independent immunoblot measurements including s.d. The fifth bar shows the Δ knd1 /WT ratio of Skp1p quantified by LC-MS/MS. Skp1p was immunopurified independently four times from 1:1 mixtures of 15 N (WT) and 14 N (Δ knd1 ) labelled cells. The average ratio and the s.d. were plotted. The sixth bar shows the average ratio of all proteins identified in the Skp1p purification. The ratio of these background proteins was close to 1.0 with a narrow s.d., supporting the significance of the ~1.5-fold increase in Skp1p levels in Δ knd1 cells. ( c ) Schematic outline of the 15 N pulse labelling strategy. Cells maintained in routine 14 N media were shifted to 15 N media for 120 or 240 min before the preparation of cell lysate, Cul1p IP and analysis by LC-MS/MS. ( d ) Relative fractions of newly synthesized FBPs and COP9 signalosome (CSN) subunits associated with Cul1p in wild-type and Δ knd1 cells. Data represent averages and s.d. values of three independent experiments (see Supplementary Data 4 ). Full size image CAND1/Knd1p regulates CRL1 dynamics To determine how the CRL1 repertoire of cells lacking CAND1/Knd1p could be disturbed in the presence of stable amounts of core components and FBPs, we developed a metabolic 15 N pulse-labelling assay that allowed us to assess CRL1 complex dynamics. Wild-type and Δ knd1 cells were maintained in 14 N medium and then switched to 15 N medium for 120 min, followed by lysate preparation, Cul1p immunopurification and LC-MS/MS analysis of the retrieved proteins ( Fig. 2c ). As we had previously shown that CAND1/Knd1p does not affect FBP stability [12] , changes in the 14 N/ 15 N peptide ratios of CRL1 components inform primarily on the rate with which newly synthesized components become assembled into CRL1 complexes in wild-type cells relative to Δ knd1 cells. Performing this experiment in triplicate, we found a statistically significant diminution in the incorporation of Skp1p and several FBPs into CRL1 complexes ( Fig. 2d , Supplementary Data 4 ). The observation was confirmed in an independent experiment in which the pulse labelling was performed for 240 min ( Supplementary Fig. S2 ; Supplementary Data 5 ). Slow incorporation of newly synthesized FBP may occur because pre-existing CRL1 complexes are stabilized in the absence of knd1 . We tested this prediction in an in vivo competition experiment. We perturbed steady-state CRL1 complexes by expressing from a plasmid Myc epitope-tagged Pof15p. This FBP is severely depleted from CRL complexes in Δ knd1 cells ( Fig. 1b , Supplementary Table S1 ), indicating that it requires Knd1p to successfully compete for CRL1 core subunits. Pof15p was expressed in a strain that harbours endogenously tagged Pof10p-Myc, an FPB that strongly accumulates in CRL1 complexes in Δ knd1 cells ( Fig. 1b , Supplementary Table S1 ). The strains were constructed in two backgrounds, wild-type and Δ knd1 . Myc-Pof15p expression was turned on and CRL1 complexes were immunoprecipitated after different times and monitored for the levels of co-precipitated Pof10p-Myc. We found that a ~10-fold excess of exogenous Pof15p efficiently displaced Pof10p-Myc from Cul1p ( Fig. 3a ). This competition was completely abolished by disrupting the F-box motif of Pof15p, confirming that it is not an indirect effect of overexpressing Pof15p ( Supplementary Fig. S3 ). Importantly, the displacement of Pof10p-Myc from Cul1p by the competing Pof15p was drastically reduced in the absence of Knd1p even though Pof15p accumulated more readily upon overexpression in Δ knd1 cells ( Fig. 3a ). The inefficiency of Pof15p in competing off Pof10p from Cul1p in the absence of Knd1p suggests that Pof15p is compromised in assembling into a CRL1 complex. Indeed, Pof15p expressed at low, non-competing levels in wild-type and Δ knd1 cells was less efficiently recruited into a complex with Cul1p when Knd1p was missing ( Fig. 3b ). Thus, CAND1/Knd1p appears to assist in CRL1 assembly by destabilizing pre-existing Cul1p-FBP interactions thereby making Cul1p available for engagement in new CRL1 complexes. 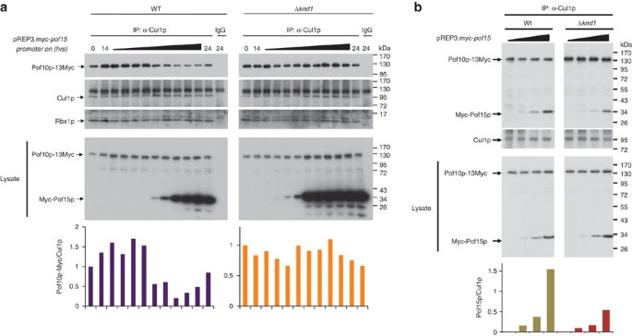Figure 3: CRL1 complexes are stabilized in the absence of Knd1p. (a) Myc epitope-tagged Pof15p was expressed from a pREP3 plasmid containing an inducible promoter in strains that harbour endogenously tagged Pof10p-Myc. The strains were constructed in two backgrounds, wild-type (WT) and Δknd1. Myc-Pof15p expression was switched on by the removal of thiamine for 14–24 h as indicated. CRL1 complexes were immunoprecipitated with anti-Cul1p antibodies and monitored for the levels of co-precipitated Pof10p-Myc and Myc-Pof15p. As a specificity control, the 24-h lysate was used for immunoprecipitation with rabbit IgG. The level of Pof10p bound to Cul1p was quantified and plotted in a bar chart. The bottom panel shows total lysates. (b) Same experiment as ina,but with Myc-Pof15p expressed at low, non-competing levels. The level of Pof15p bound to Cul1p was quantified and plotted in a bar chart. Figure 3: CRL1 complexes are stabilized in the absence of Knd1p. ( a ) Myc epitope-tagged Pof15p was expressed from a pREP3 plasmid containing an inducible promoter in strains that harbour endogenously tagged Pof10p-Myc. The strains were constructed in two backgrounds, wild-type (WT) and Δ knd1 . Myc-Pof15p expression was switched on by the removal of thiamine for 14–24 h as indicated. CRL1 complexes were immunoprecipitated with anti-Cul1p antibodies and monitored for the levels of co-precipitated Pof10p-Myc and Myc-Pof15p. As a specificity control, the 24-h lysate was used for immunoprecipitation with rabbit IgG. The level of Pof10p bound to Cul1p was quantified and plotted in a bar chart. The bottom panel shows total lysates. ( b ) Same experiment as in a, but with Myc-Pof15p expressed at low, non-competing levels. The level of Pof15p bound to Cul1p was quantified and plotted in a bar chart. Full size image CAND1 displaces FBPs from Cul1p in vitro To further test this idea, we asked whether recombinant CAND1 could displace FBPs from Cul1p. Cul1p complexes were immunopurified and incubated with recombinant human CAND1 ( Supplementary Fig. S4a ) for 30 min followed by measuring the amount of Pof10p-Myc retained in the complex. In a reciprocal experiment, Pof10p-Myc complexes were purified and incubated with CAND1. In both experiments, CAND1 led to an apparent release of Pof10p from Cul1p ( Fig. 4a ). The same activity of CAND1 was observed for Pof1p-Myc complexes ( Supplementary Fig. S4b ). A kinetic experiment showed that the FBP releasing activity of CAND1 depended on its ability to bind Cul1p, as fully neddylated Cul1p complexes isolated from Δ knd1 Δ csn5 cells were largely resistant to CAND1-mediated FBP release ( Fig. 4b ). The minor release of Pof10p that occurred after 100 min of incubation with CAND1 is consistent with the recent observation that neddylated Cul1p retains a minimal ability to interact with CAND1 (ref. 30 ). Lack of the release activity of CAND1/Knd1p may thus cause the increased stability of Cul1p-FBP interactions observed in vivo . 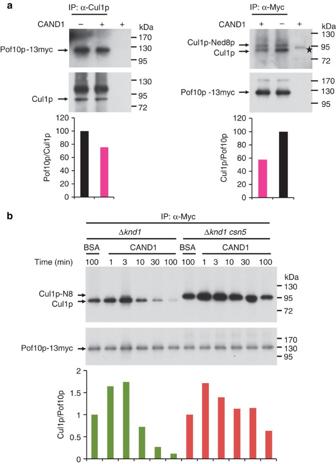Figure 4: CAND1 displaces F-box proteins from Cul1p. (a) Cul1p- and Pof10p-associated protein complexes were immunopurified from Δknd1cells and incubated with 1 μg of recombinant His-tagged human CAND1 for 30 min. One microgram of bovine serum albumin was used as control instead of CAND1. The complexes were analysed for the levels of Cul1p and Pof10p-Myc by immunoblotting with Cul1p and Myc antibodies, and signals were quantified. The asterisk denotes a band present in the CAND1 preparation that weakly crossreacts with the α-Cul1p antiserum (possibly insect cell CUL1). (b) Pof10p-Myc complexes were isolated from Δknd1and Δknd1 csn5cells as in (a) and incubated for the indicated times with 1 μg BSA or CAND1 as indicated. The complexes were analysed for the levels of Cul1p and Pof10p-Myc by immunoblotting with Cul1p and Myc antibodies, and signals were quantified. Figure 4: CAND1 displaces F-box proteins from Cul1p. ( a ) Cul1p- and Pof10p-associated protein complexes were immunopurified from Δ knd1 cells and incubated with 1 μg of recombinant His-tagged human CAND1 for 30 min. One microgram of bovine serum albumin was used as control instead of CAND1. The complexes were analysed for the levels of Cul1p and Pof10p-Myc by immunoblotting with Cul1p and Myc antibodies, and signals were quantified. The asterisk denotes a band present in the CAND1 preparation that weakly crossreacts with the α-Cul1p antiserum (possibly insect cell CUL1). ( b ) Pof10p-Myc complexes were isolated from Δ knd1 and Δ knd1 csn5 cells as in ( a ) and incubated for the indicated times with 1 μg BSA or CAND1 as indicated. The complexes were analysed for the levels of Cul1p and Pof10p-Myc by immunoblotting with Cul1p and Myc antibodies, and signals were quantified. Full size image CAND1/Knd1p is required for efficient substrate degradation Our data suggested an important role for CAND1/Knd1p in organizing the cellular CRL1 repertoire such as to optimize substrate degradation. To test this, we assessed the impact of Knd1p on the degradation of the CRL1 Pof3p substrate Ams2p (ref. 31 ). Similar to what we describe for CRL1 complexes containing Pof5p, Pof11p and Pof15p in Fig. 1b , the level of CRL1 Pof3p is ~50% diminished in Δ knd1 cells [12] . Consistent with this downregulation, we found a ~2-fold upregulation of the steady-state levels of Ams2p in Δ knd1 cells, which coincided with an increase in half-life ( Fig. 5a ). Similar to Δpof3 cells, which accumulate Ams2p (ref. 24 ), we found Δ knd1 cells to be sensitive to the genotoxic replication inhibitor hydroxyurea ( Fig. 5b ). CAND1/Knd1p-mediated maintenance of the CRL1 landscape, therefore, appears critical for substrate degradation and normal physiology. 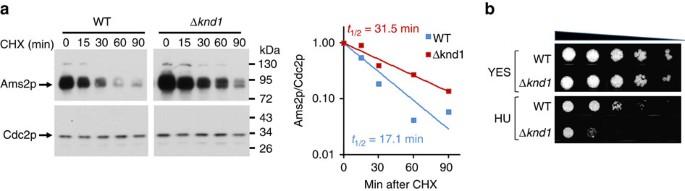Figure 5: Knd1p is required for efficient CRL1-mediated substrate degradation. (a) Wild-type and Δknd1cells were incubated with 100 μg ml−1cycloheximide (CHX) for the indicated times and Ams2p levels were determined by immunoblotting relative to the loading control Cdc2p. The graph on the right shows a quantification of the results. Exponential trend lines were fitted through the data points in Excel, and the resulting equations were used to calculate half-lives. (b) Hydroxyurea sensitivity of Δknd1cells. Fivefold serial dilutions of wild-type and Δknd1cells were spotted onto media with (bottom) or without (top) 10 mM hydroxyurea. Figure 5: Knd1p is required for efficient CRL1-mediated substrate degradation. ( a ) Wild-type and Δ knd1 cells were incubated with 100 μg ml −1 cycloheximide (CHX) for the indicated times and Ams2p levels were determined by immunoblotting relative to the loading control Cdc2p. The graph on the right shows a quantification of the results. Exponential trend lines were fitted through the data points in Excel, and the resulting equations were used to calculate half-lives. ( b ) Hydroxyurea sensitivity of Δ knd1 cells. Fivefold serial dilutions of wild-type and Δ knd1 cells were spotted onto media with (bottom) or without (top) 10 mM hydroxyurea. Full size image Our data obtained by complete genetic ablation of CAND1 suggest a novel function of CAND1/Knd1p in controlling the in vivo dynamic exchange of FBPs from Cul1p. We propose that lack of this activity ‘freezes’ FBP exchange. Therefore, in the presence of stable but limiting amounts of Cul1p, those CRL1 complexes that are formed by FBPs that have relatively higher intrinsic ratios of on-rate/off-rate for Cul1p would out-compete those formed by FBPs with lower ratios. In addition, the degradation rates of individual FBPs may vary and, in the absence of CAND1/Knd1p, FBPs that turn over more quickly would become progressively displaced by those that are more stable thus leading to the observed imbalances. These imbalances may augment the degradation of substrates of CRL1 complexes that accumulate in the absence of CAND1/Knd1p while at the same time curtailing the destruction of substrates of those CRL1 ligases that are depleted. The CRL1 Pof3p substrate Ams2p is one such example. This interpretation can reconcile conflicting reports of simultaneous positive as well as negative effects of CAND1 depletion on CRL-mediated substrate degradation in vivo [32] . The proposition that CAND1/Knd1p functions transiently as a FBP exchange factor can rationalize our previous observation that only a very small fraction of Knd1p is in a stable complex with Cul1p (ref. 12 ), a finding that was subsequently confirmed in human cells [27] . This finding combined with the data on CRL dynamics and our demonstration that CAND1 can displace FBPs from Cul1p in vitro strongly suggest that CAND1 drives a cycle of continuous and rapid FBP recruitment and displacement which we dubbed the ‘CAND1 cycle’ [12] . This cycle would provide the dynamicity that assures comprehensive sampling of the steady-state FBP repertoire. Our data, therefore, qualify the conclusion of a previous study that CRL network organization is driven by the abundance of FBPs but not by cycles of CAND1 binding and release [27] . Rather, we argue that CAND1/Knd1p accounts for the activity that assures that the CRL1 repertoire is a reflection of the steady-state abundance of FBPs. These considerations also resolve the surprising observation that the CRL1 repertoire is not greatly disturbed when CUL1 neddylation is pharmacologically inhibited by MLN4924 [27] , [33] because CAND1-mediated equilibration of FBPs would continue to operate—and in fact would be predicted to be more efficient—in the absence of neddylation. From our studies, the general principle arises that the problem of substrate receptor competition that is inherent to the vast combinatorial architecture of CRLs is solved through the coordinated interplay of the CAND1 cycle with the neddylation/deneddylation cycle. For a given molecule of CUL1, the CAND1-mediated continuous substrate receptor exchange cycle would be interrupted only upon neddylation. As substrate can stimulate cullin neddylation [19] , [30] , [34] , CRLs containing receptors fitting a particular substrate that is present at a certain point in time would be selectively removed from the CAND1 cycle and thus activated. Upon substrate consumption, substrate receptors likely succumb to autocatalytic destruction or are recycled [11] , [35] . COP9 signalosome-mediated deneddylation would re-enter these complexes into the CAND1 cycle. In this scenario, which is consistent with in vitro data [18] , [19] as well as our study on in vivo CRL dynamics, CAND1 would function as a substrate receptor exchange factor that accelerates the approach of the unneddylated CRL1 repertoire to equilibrium. Interestingly, CAND1 was originally identified as a factor that stimulates the integration of RNA polymerase II/TFIIF into the TFIID-TFIIB-DNA-complex [36] , raising the intriguing possibility that CAND1 may also promote the dynamics of other large protein complexes that require the same high degree of dynamicity as CRLs. 15 N stable isotope labelling and immunopurification of CRL1 The yeast strains used in this study are summarized in Supplementary Table S2 . For stable isotope labelling, cells lacking any nutritional markers were grown at 30 °C for 10 generations on Edinburgh minimal medium (EMM) plates containing either ammonium- 14 N chloride (strain SDW542/2, cul1-13myc:kan knd1::ura4 ) or ammonium- 15 N chloride (strain SDW542/1, cul1-13myc:kan ) as the nitrogen sources. 15 N labelling efficiency was at least 98% as determined by mass spectrometry. For immunopurification of CRL1 complexes, cells were grown to optical density (OD) 600nm ~1.0 in 1,000 ml EMM supplemented with the respective light or heavy ammonium chloride. Cells were harvested by centrifugation and washed with STOP buffer (150 mM NaCl, 10 mM EDTA, 50 mM NaF, 1 mM NaN 3 ) once and flash frozen in liquid nitrogen. Equal amounts of wild-type and Δ knd1 mutant cells were mixed and disrupted by bead lysis in 14 ml immunoprecipitation buffer (25 mM Tris-HCl pH 7.5, 50 mM NaCl, 0.1% Triton X100, 1 mM phenylmethyl sulphonyl fluoride (PMSF), 5 μg ml −1 aprotinin, 10 μg ml −1 leupeptin, 10 μg ml −1 pepstatin). Cell lysates were cleared by centrifugation at 18,000 r.p.m. and subjected to immunoprecipitation with 300 μl pre-equilibrated anti-c-Myc agarose (Clontech, cat no. 631208) for 2 h. Beads were washed and eluted with 200 μl of 100 mM glycine, pH 2.0 and neutralized with 20 μl of 2 M Tris-HCl, pH 9.0. Five percent of the eluate was loaded onto a gel to estimate the protein amount. The remainder was analysed by LC-MS/MS. Pulse labelling with 15 N Wild-type (SDW542/1) and Δ knd1 mutant cells (SDW542/2) were grown to OD 600nm ~1.0 in 1,000 ml EMM containing ammonium- 14 N chloride (light medium) at 30 °C. Cells were harvested by centrifugation and transferred to 1,000 ml of EMM containing ammonium- 15 N chloride (heavy media). After labelling periods of 120 or 240 min, cells were harvested by centrifugation and washed with STOP buffer once and frozen in liquid nitrogen. Cell lysis and affinity purification of CRL1 complexes was as described above. One-dimensional LC-MS/MS Immunopurified protein complexes were first reduced and alkylated using Tris (2-carboxyethyl) phosphine hydrochloride and iodoacetamide, then digested using Trypsin as previously described in detail [37] . After desalting, the peptides were analysed by reverse-phase LC-MS/MS, using a Michrom Paradigm high-performance liquid chromatography with a Magic C18 column and a LTQ-Orbitrap XL mass spectrometer (Thermo-Fisher). The peptides were separated on a 120-min gradient of 10–30% buffer B (100% acetonitrile/0.1% formic acid). Tandem mass spectrometry (MS/MS) spectra were collected during the LC-MS runs. Each scan was set to acquire a full MS scan, followed by MS/MS scans on the four most intense ions from the preceding MS scan. To maximize coverage, each IP sample was analysed by LC-MS/MS three times (technical replicates). Data analysis and protein quantification Both protein identification and quantification of isotopically labelled peptides/proteins were performed by IP2, a comprehensive programme package including SEQUEST, ProLuCID, DTASelect and Census (Integrated Proteomics Applications Inc., San Diego, CA, USA). First, MS1 and MS2 files were extracted by RawExtract (The Scripps Research Institute, La Jolla, CA, USA) from the raw LC-MS/MS spectra obtained on the LTQ-Orbitrap XL. Then a Swissprot S. pombe protein database was uploaded into IP2, which automatically generated a reverse decoy protein database. The MS1 and MS2 files of the three technical replicates of each sample were uploaded to IP2 server, and the combined MS1 and MS2 files were searched using ProLuCID and the decoy database. Differential modification included 16 Da on methionine for oxidation. The identification results from ProLuCID were filtered and organized by DTASelect. The DTASelect parameters were carefully set so that the false-positive rate of protein identification was below 1.5%. The heavy and light spectral counts were obtained for each protein after ProLuCID/DTASelect analysis. Finally the quantification analysis was selected for 15 N. Protein ratios and s.d. values were calculated by Census (based on peptides with a factor of determination of ≥0.5). 15 N enrichment of each sample was calculated by IP2 as well and found to be at least 98%. Protein quantifications with high s.d. values for individual peptides or low peptide numbers were manually examined, and outliers were removed if necessary. To adjust for slight differences in 15 N labelling efficiency in short-term experiments, the protein ratios in the pulse labelling samples were normalized to the average ratio of all proteins quantified in the corresponding sample from wild-type cells. Average protein ratios were averaged over multiple replicates and s.d. values and P -values were calculated. To obtain robust data sets, quantifications with a relative s.d.>35% were excluded from the final data. AQUA of CRL1 components by LC-MS/MS Based on our LC-MS/MS analysis of tryptic digests, we selected peptides TFFETNFIENTK, ELADDDVIWHR, TGVSLQSFQFR and LSFLDEYSLR as AQUA standard peptides for Cul1p, Pof1p, Pof10p and Pof15p, respectively. The AQUA peptides were purchased from Thermo-Fisher and Sigma-Aldrich, with stable isotopes ( 13 C, 15 N) in the C-terminal lysine or arginine. As the AQUA reference peptides are isotopically distinct from their corresponding endogenous 14 N and 15 N peptides, we can quantify both ‘light’ and ‘heavy’ proteins in a single analysis of immunopurified CRL1 complexes isolated from 15 N or 14 N-labelled cells. An LTQ-Orbitrap method was developed that performs selected ion monitoring followed by MS/MS confirmation of the peptides. A quantity of 100 fmol of the standard peptides was spiked into the digests of CRL1 complexes immunopurified from a 1:1 mixture of wild-type and Δ knd1 cell lysate. The peptides were separated by the same 120 min gradient LC method on the same LC-LTQ Orbitrap XL system as used for peptide identification. During the AQUA analysis, selected ion monitoring spectra were first collected in the 630–760 m/z range with 60,000 Fourier transform mass spectrometry (FTMS) resolution, followed by MS/MS scans of the nine peptide ions with known m/z. Peak integrations were obtained through the application of extracted ion chromatograms over 10-p.p.m. mass intervals on Qual Browser (Thermo-Fisher). No contaminating peptides were found to coelute with the four peptides chosen for Cul1p, Pof1p, Pof10p and Pof15p. The analysis was repeated five times. Raw data for a representative AQUA experiment are shown in Supplementary Fig. 5 . Hydroxyurea sensitivity assay Fivefold serial dilutions of wild-type (SDW542/1) and Δ knd1 mutant (SDW542/2) cells were spotted onto control YES plates or plates containing 10 mM hydroxyurea. Plates were incubated at 30 °C for 5 days. FBP competition experiment The pof15 (SPAPB1A10.14) gene was cloned into the vector pREP3-6His.Myc, which drives the expression of N-terminal 6His-Myc-tagged protein from the thiamine repressible nmt1 promoter. A Pof15p mutant lacking residues 34–40 (LPVEVID) within the F-box motif was generated in the same expression vector. The plasmid were confirmed by sequencing and transformed into wild-type and Δ knd1 mutant cells harbouring a Myc-tagged allele of pof10 at the endogenous genomic locus ( pof10-13myc ). The expression of pof15 was induced by removal of thiamine from the culture medium for increasing periods of time followed by preparation of cell lysates by bead lysis in immunoprecipitation buffer ( 25 mM Tris-HCl pH 7.5, 50 mM NaCl, 0.1% Triton X100, 1 mM PMSF, 5 μg ml −1 aprotinin, 10 μg ml −1 leupeptin, 10 μg ml −1 pepstatin). Lysates were subjected to immunoprecipitation with rabbit anti-Cul1p antibody [38] , followed by collection of immunocomplexes on protein A Sepharose beads (Rockland, cat no. PA50-00-0005). The immunoprecipitated complexes were analysed by immunoblotting. Myc-tagged FBPs were detected with a monoclonal anti-Myc antibody (9E10, cat. no. 13-2500, Invitrogen). Expression and purification of recombinant human CAND1 The CAND1 isoform 1 open reading frame was PCR amplified from the MegaMan Human Transcriptome library (Agilent) with 3′-sequences encoding a hexahistidine tag immediately 5′ of the stop codon and used to generate a recombinant baculovirus using the FastBac system (Invitrogen). After 48 h of infecting Hi5 insect cell cultures (10e8 cells) at a multiplicity of infection >10, CAND1 was purified by Ni-NTA chromatography and desalted into 25 mM HEPES pH 7.6, 100 mM NaCl and 10% glycerol. FBP displacement assay with recombinant CAND1 Cells harbouring endogenous Pof10p modified with Myc epitopes were grown to an OD 600nm of ~1.0 in 200 ml of YES. Cell lysates were prepared by beads lysis in immunoprecipitation buffer (25 mM Tris-HCl pH 7.5, 50 mM NaCl, 0.1% Triton X100, 1 mM PMSF, 5 μg ml −1 aprotinin, 10 μg ml −1 leupeptin, 10 μg ml −1 pepstatin). Pof10p was immunopurified on pre-equilibrated anti-c-Myc agarose beads (Clontech, cat. no. 631208). In a reciprocal experiment, Cul1p complexes were immunoprecipitated with Cul1p antibodies. The complexes were washed and divided into two aliquots. One microgram of recombinant His-tagged human CAND1 expressed in and purified from insect cells was added to one aliquot and incubated at 30 °C for 30 min. One microgram of bovine serum albumin was used as control instead of CAND1. After washing, the immunoprecipitated complexes were analysed by immunoblot. Myc-tagged protein was detected with monoclonal anti-c-Myc antibody (9E10, cat. no. 13-2500, Invitrogen), and Cul1p with rabbit anti-Cul1p antibody. Immunoprecipitation and immunoblotting of CRL1 complexes Cell lysates for immunoprecipitation of Myc-tagged FBPs were prepared as described in a buffer containing 50 mM Tris, pH 7.4, 50 mM NaCl and 0.5% Triton X100 (ref. 12 ). Lysates were cleared by centrifugation, and proteins were precipitated with the respective antisera (anti-Myc, anti-Rbx1p). Immunocomplexes were collected by binding to protein A beads, washed and analysed by immunoblotting. Affinity-purified rabbit antisera against Cul1p, Skp1p and Rbx1p were described previously [38] , [39] . Ams2p antisera were kindly provided by Y. Takayama [31] . For loading controls Cdc2p (PSTAIRE, Santa Cruz) antibodies were used at a dilution of 1:500. How to cite this article: Wu, S. et al . CAND1 controls in vivo dynamics of the Cullin 1-RING ubiquitin ligase repertoire. Nat. Commun. 4:1642 doi: 10.1038/ncomms2636 (2013).